Glycan clustering stabilizes the mannose patch of HIV-1 and preserves vulnerability to broadly neutralizing antibodies The envelope spike of HIV-1 employs a ‘glycan shield’ to protect itself from antibody-mediated neutralization. Paradoxically, however, potent broadly neutralizing antibodies (bnAbs) that target this shield have been isolated. The unusually high glycan density on the gp120 subunit limits processing during biosynthesis, leaving a region of under-processed oligomannose-type structures, which is a primary target of these bnAbs. Here we investigate the contribution of individual glycosylation sites in the formation of this so-called intrinsic mannose patch. Deletion of individual sites has a limited effect on the overall size of the intrinsic mannose patch but leads to changes in the processing of neighbouring glycans. These structural changes are largely tolerated by a panel of glycan-dependent bnAbs targeting these regions, indicating a degree of plasticity in their recognition. These results support the intrinsic mannose patch as a stable target for vaccine design. The envelope spike of HIV-1 (Env) orchestrates host cell entry and is the primary target for neutralizing antibodies. Env is a heavily glycosylated molecule, with N-linked glycans accounting for approximately half of the mass of gp120 (ref. 1 ). These glycans provide essential roles in protein folding and infectivity [2] , [3] and also act to shield the underlying protein epitopes from recognition by neutralizing antibodies [4] . The N-linked glycans of gp120 are synthesized using the host cell glycosylation machinery. However, characterization of the glycoforms present has identified a significant population of unprocessed oligomannose-type glycans on gp120, termed the intrinsic mannose patch, which are not usually observed at high abundance on secreted mammalian glycoproteins [5] , [6] , [7] , [8] . This divergence from host cell glycosylation is thought to derive from the exceptionally high density of glycans on the outer domain of gp120, which restricts access to the endoplasmic reticulum (ER) and Golgi α-mannosidases and prevents the subsequent processing reactions that typically lead to synthesis of complex-type glycans [7] . The ‘non-self’ nature of these oligomannose glycans suggests they could represent a potentially immunogenic target, and indeed a number of broadly neutralizing anti-HIV-1 antibodies (bnAbs) have been isolated that incorporate gp120 glycans as part of their epitope [9] , [10] , [11] , [12] . 2G12 was the first such antibody to be described, which exploits an unusual domain-exchanged configuration and binds terminal Manα1→2Man residues on the surface of gp120 (refs 13 , 14 , 15 ). More recently, a collection of bnAbs has been described that recognize dual protein-glycan epitopes [9] , [11] , [12] , [16] , [17] , [18] , [19] , [20] , [21] , [22] , [23] , [24] , [25] . A number of these, including PGT121, PGT128 and PGT135, have been demonstrated to be dependent on the outer domain glycan at N332, with this site being referred to as a ‘supersite’ of immune vulnerability [9] , [17] , [19] , [26] , [27] . Comparison of these bnAbs with those targeting alternative epitopes on gp120, including the CD4-binding site (CD4bs) or membrane-proximal external region (MPER), reveal that they offer some of the highest potencies of neutralization [9] . Furthermore, the different bnAbs derive from various combinations of antibody germline genes, indicating that there are multiple solutions for targeting this region [9] , [20] , [27] . Passive transfer of such bnAbs confers resistance to viral challenge in macaque studies [29] , [30] , [31] , and thus efforts are being focused to elucidate their precise epitopes, with the aim of designing immunogens capable of eliciting such neutralizing responses through vaccination [32] . However, a concern regarding the targeting of gp120 glycans relates to the shifting nature of the glycan shield, with additions and deletions of glycan sites being a common response by HIV-1 to antibody-mediated selection pressure [33] , [34] . Here we investigate the integrity and robustness of the oligomannose population of gp120 in the face of sequence variation, and determine the consequences of glycan site mutation on the formation of bnAb epitopes. Systematic site-directed mutagenesis of the potential N-glycosylation sites (PNGSs) of gp120 BaL demonstrates widespread conservation of the oligomannose population, although unexpectedly large perturbations are observed upon loss of certain PNGSs. Structural modelling of the glycan shield reveals protein–glycan and glycan–glycan packing that suggests an explanation for these observations and rationalizes the characteristic processing observed at different glycosylation sites. While it is demonstrated that mutation of sites involved in glycan clusters can lead to subtle ‘bystander’ processing effects, these changes can largely be tolerated by a panel of bnAbs. The conservation and persistence of oligomannose-type glycans, despite glycan site deletion, suggests that the intrinsic mannose patch is likely to be an important component of an effective vaccine. Resilience of the mannose patch to glycan site deletion Site-specific glycosylation analysis of recombinant gp120 indicates that, depending on the isolate, up to half of the PNGSs are occupied by oligomannose-type glycans [1] , [5] , [6] , [35] , [36] , [37] . Given the perceived role of glycan density in driving the formation of the intrinsic mannose patch, it is conceivable that the loss of a single glycan could have a widespread effect on many near and distant glycans by changing the processing state of its neighbours. In this scenario, glycans that would otherwise be protected by a neighbouring glycan become exposed and are processed by cellular enzymes to complex-type structures. We therefore sought to investigate the role of an individual glycan site in the formation of the intrinsic mannose patch by site-directed mutagenesis of all 23 gp120 PNGSs of the clade B isolate, BaL. Asparagine residues within the consensus sequence Asn-X-Ser/Thr (where X is any amino acid except Pro) were mutated to alanine. The gp120 constructs were then expressed transiently in 293T cells and purified by nickel affinity chromatography. Expression of the panel of gp120 BaL mutants was performed in parallel to minimize the intrinsic variation of glycosylation ( Supplementary Fig. 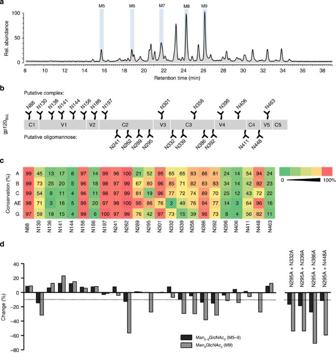Figure 1: Contribution of individual glycans to the total glycosylation of gp120BaL. (a) HILIC-UPLC profile of N-linked glycans released from gp120BaL. The Man5-9GlcNAc2series is labelled M5–M9 and highlighted in blue. Remaining peaks correspond to hybrid- and complex-type glycans. (b) Schematic showing the distribution of the 23 PNGSs of gp120BaL. Sites were allocated as putative complex-type or putative oligomannose-type based on previous reports1,35,36,37. (c) Percentage conservation of the individual PNGSs across different clades, based on analysis of over 4,000 aligned Env sequences from the Los Alamos HIV sequence database (http://www.hiv.lanl.gov/). (d) Effect of PNGS-deletion on the total abundance of oligomannose-type glycans, and the individual abundance of Man9GlcNAc2. Values were obtained by integration of corresponding HILIC-UPLC peaks (Supplementary Fig. 2), before and after Endoglycosidase H treatment, and represent the percentage change in abundance (relative to wild-type). Percentage change=[(% oligomannose in wild-type−% oligomannose in mutant)/(% oligomannose in wild-type)] × 100. Values are reported inSupplementary Table 2. The dashed line represents the predicted drop in oligomannose levels from the elimination of one site containing only oligomannose-type glycans. 1 ; Supplementary Table 1 ). Following resolution by sodium dodecyl sulfate–PAGE (SDS–PAGE), N-linked glycans were released from monomeric gp120 by treatment with protein N -glycosidase F (PNGase F) and analysed by hydrophilic interaction liquid chromatography-ultra performance liquid chromatography (HILIC-UPLC). HILIC-UPLC was used as it offers a quantitative method for analysis of complex glycan mixtures that is not biased by the glycan composition. Integration of the HILIC-UPLC spectra together with digestions of the fluorescently labelled glycan pool with Endo H enabled the quantitation of oligomannose species. The HILIC-UPLC chromatogram of the glycans from wild-type gp120 BaL reveals a mixture of complex- and oligomannose-type glycans ( Fig. 1a ). Many of the glycosylation sites on gp120 BaL predicted to be of the oligomannose-type [1] , [35] , [37] , [38] ( Fig. 1b ) show a high degree of conservation across different clades ( Fig. 1c ). Changes in the total abundance of oligomannose-type glycans (relative to wild-type) were calculated from the HILIC-UPLC data ( Fig. 1d ; Supplementary Fig. 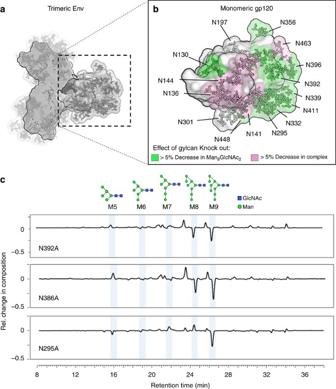Figure 2: Role of glycan clusters in maintaining the oligomannose population. (a) Model of a fully glycosylated BaL trimer based on the reported gp140 trimer crystal structure21(PDB accession code: 4NCO). Modelled glycans are shown as sticks. The surface of the glycans and underlying protein are depicted in shades of grey. Man5GlcNAc2glycans were modelled at sites of predicted complex-type glycans and Man8GlcNAc2glycans were added at predicted oligomannose sites. (b) A close-up view of the gp120 monomer. Glycans are coloured according to the effect of their elimination on total Man9GlcNAc2levels or complex-type glycosylation according toFig. 1d. A change of over 5% is greater than the intrinsic variation of glycosylation (Supplementary Fig. 1;Supplementary Table 1). (c) Examples of changes in glycan composition upon deletion of individual glycan sites of the mannose patch. Residual plots were calculated by the subtraction of HILIC-UPLC spectra of PNGS-deletion mutants from that of the wild-type. Peaks corresponding to oligomannose-type glycans are highlighted. Man5-9GlcNAc2(M5–9) are schematically labelled according to the combined nomenclature69of Harveyet al.70and the Center of Functional Glycomics. 2 ; Supplementary Table 2 ). Overall, the direction of change corresponded well with the predicted glycan species at each site; loss of predicted complex sites showed an increased relative abundance of oligomannose-type glycans, while loss of predicted sites of oligomannose generally resulted in lower relative abundances of oligomannose-type glycans. For a few PNGS-deletions, for example, N386 and N392, larger than expected losses of oligomannose were observed (14 and 15% decreases, respectively). These PNGSs may represent sites that normally impede the access of α-mannosidases to neighbouring sites, whereby their removal facilitates greater access and trimming of surrounding glycans. Figure 1: Contribution of individual glycans to the total glycosylation of gp120 BaL . ( a ) HILIC-UPLC profile of N-linked glycans released from gp120 BaL . The Man 5-9 GlcNAc 2 series is labelled M5–M9 and highlighted in blue. Remaining peaks correspond to hybrid- and complex-type glycans. ( b ) Schematic showing the distribution of the 23 PNGSs of gp120 BaL . Sites were allocated as putative complex-type or putative oligomannose-type based on previous reports [1] , [35] , [36] , [37] . ( c ) Percentage conservation of the individual PNGSs across different clades, based on analysis of over 4,000 aligned Env sequences from the Los Alamos HIV sequence database ( http://www.hiv.lanl.gov/ ). ( d ) Effect of PNGS-deletion on the total abundance of oligomannose-type glycans, and the individual abundance of Man 9 GlcNAc 2 . Values were obtained by integration of corresponding HILIC-UPLC peaks ( Supplementary Fig. 2 ), before and after Endoglycosidase H treatment, and represent the percentage change in abundance (relative to wild-type). Percentage change=[(% oligomannose in wild-type−% oligomannose in mutant)/(% oligomannose in wild-type)] × 100. Values are reported in Supplementary Table 2 . The dashed line represents the predicted drop in oligomannose levels from the elimination of one site containing only oligomannose-type glycans. Full size image Thus, while some mutations led to larger than expected losses in oligomannose, the majority of PNGS-deletions had a very limited impact on the size of the mannose patch. Several double PNGS-deletion mutants were also analysed. No marked decreases in the overall abundance of oligomannose were observed, with the N295A/N386A double mutant showing the largest effect with a loss of 27% ( Fig. 1d ; Supplementary Table 2 ). As the BaL isolate lacks the N160 and N276 glycans, which are highly conserved and have been shown to be important for recognition by several bnAbs [9] , [16] , [39] , we also assessed the impact of these glycans by introducing them into the wild-type BaL sequence. These glycans were found to have a limited impact on the size of the mannose patch, either individually or when combined ( Supplementary Table 2 ). Overall these data demonstrate the stability of the size of the mannose patch in the face of glycan site deletion. Glycan–glycan interactions restrict glycan processing While the overall size of the mannose patch remained relatively unperturbed upon deletion of individual PNGSs, closer inspection of the HILIC-UPLC traces revealed that the abundances of the individual oligomannose species (Man 5-9 GlcNAc 2 ) varied more considerably. Figure 1d shows the change in levels of Man 9 GlcNAc 2 , which displayed the greatest sensitivity to removal of PNGSs ( Fig. 1d ; Supplementary Table 2 ). A decrease of over 25% was observed for nine sites: N130, N262, N295, N339, N356, N386, N392 and N448. These contrasting effects on the overall abundance of oligomannose and Man 9 GlcNAc 2 alone can be reconciled by the changing proportions of the other oligomannose species. For example at the N295 site no change in the overall level of oligomannose was detectable; however, a large decrease in Man 9 GlcNAc 2 was apparent. This decrease in Man 9 GlcNAc 2 was offset by an increase in Man 6-8 GlcNAc 2 , suggesting a redistribution of oligomannose species across the intrinsic mannose patch that goes beyond a simple loss of glycans from the N295 site. The apparent redistribution of glycoforms upon PNGS-deletion, from larger oligomannose-type glycans to smaller oligomannose species, indicates that individual PNGSs have a role in influencing the processing of glycans at neighbouring sites. To understand this phenomenon at the structural level, a model of a fully glycosylated gp120 BaL trimer was constructed based on the crystal structure of a BG505 SOSIP.664 gp140 trimer [21] ( Fig. 2a ). Man 8 GlcNAc 2 glycans were incorporated at sites of predicted oligomannose-type glycans, while Man 5 GlcNAc 2 was chosen as a representative mid-sized glycan that is commonly found alongside complex-type glycans at gp120 glycosylation sites ( Supplementary Fig. 3 ). The glycosylated model demonstrates the uniquely high density of glycans on the surface of Env that represents a significant barrier to processing by glycosidases and glycosyltransferases. Figure 2: Role of glycan clusters in maintaining the oligomannose population. ( a ) Model of a fully glycosylated BaL trimer based on the reported gp140 trimer crystal structure [21] (PDB accession code: 4NCO). Modelled glycans are shown as sticks. The surface of the glycans and underlying protein are depicted in shades of grey. Man 5 GlcNAc 2 glycans were modelled at sites of predicted complex-type glycans and Man 8 GlcNAc 2 glycans were added at predicted oligomannose sites. ( b ) A close-up view of the gp120 monomer. Glycans are coloured according to the effect of their elimination on total Man 9 GlcNAc 2 levels or complex-type glycosylation according to Fig. 1d . A change of over 5% is greater than the intrinsic variation of glycosylation ( Supplementary Fig. 1 ; Supplementary Table 1 ). ( c ) Examples of changes in glycan composition upon deletion of individual glycan sites of the mannose patch. Residual plots were calculated by the subtraction of HILIC-UPLC spectra of PNGS-deletion mutants from that of the wild-type. Peaks corresponding to oligomannose-type glycans are highlighted. Man 5-9 GlcNAc 2 (M5–9) are schematically labelled according to the combined nomenclature [69] of Harvey et al. [70] and the Center of Functional Glycomics. Full size image Plotting of the changes in Man 9 GlcNAc 2 abundance on to the gp120 monomer defined a region of high glycan density that was sensitive to deletion of local PNGSs ( Fig. 2b ). This region mapped to the outer domain of gp120 and is consistent with previous observations of the intrinsic mannose patch [1] , [5] , [6] , [35] , [36] , [37] . Closer inspection of individual PNGSs within this region revealed sites of glycan clusters with two or more glycans positioned in very close proximity. For example, one such cluster involves the N386 and N392 glycans, in which the Asn Cα atoms are positioned ∼ 12 Å apart. Deletion of the N392 glycan led to an overall decrease in oligomannose abundance of 15% ( Fig. 1d and Supplementary Table 2 ), primarily driven by losses of Man 9 GlcNAc 2 and Man 8 GlcNAc 2 (32 and 22% relative to wild-type, respectively; Fig. 2c ). Another cluster was identified based around the N295 glycan, which occupies a central location between the N332 and N448 sites. While loss of the N295 glycan had no overall effect on the total abundance of oligomannose, it resulted in a 28% decrease in Man 9 GlcNAc 2 ( Fig. 2c ; Supplementary Table 2 ). Glycan–glycan interactions within these tight clusters not only suggest an explanation for the limited processing of these glycans, but could rationalize the more widespread changes to glycan processing observed upon removal of a single glycan. It is likely that removal of a glycan within such a cluster increases mobility and accessibility to its neighbouring glycan(s), thereby increasing the level of processing that can occur. Changes in protein conformation distort glycan processing While many of the PNGS-deletion mutants displayed modest changes in glycosylation, some displayed larger than expected differences that could not be rationalized by cluster effects. One explanation is that either the Asn→Ala mutation, or loss of the glycan, induces protein misfolding, leading to altered glycan processing. To test this possibility ELISAs were performed using b12, a CD4bs conformation-dependent antibody ( Fig. 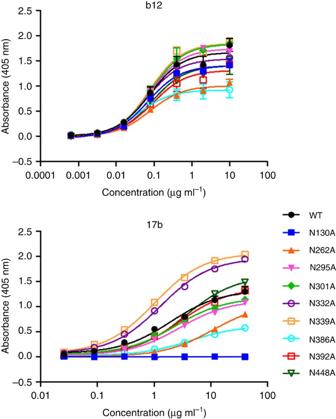Figure 3: Recognition of PNGS-deletion mutants by conformation-dependent antibodies. Binding of the conformation-dependent monoclonal antibodies b12 and 17b was tested against the panel of gp120BaLPNGS-deletion mutants by capture ELISA. Error bars represent s.d. Each experiment was performed in duplicate and repeated three times. 3 ; Supplementary Table 3 ). The binding of the majority of the PNGS-mutants was unchanged relative to wild-type, with the exception of N262A and N386A, which displayed significantly reduced binding plateaus. 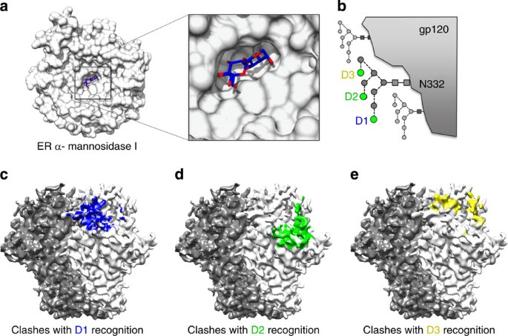Figure 4: Steric barriers to the processing of Env glycans. The α-mannosidase enzyme has impeded access to the terminal sugars of the mannose patch due to steric constraints imposed by both protein and glycan moieties. (a) The high-resolution structure of α1,2-mannosidase (PDB accession code: 2RI9) bound to a disaccharide substrate shows how the substrate binds in a deep, concave pocket. (b) When the α-1,2-mannosidase structure is docked onto the surface of the HIV-1 Env trimer (hybrid model of EMD-5779 and PDB 3TYG) and aligned on the terminal D1, D2 or D3 arms of the Man9GlcNAc2moiety at position N332, there are significant clashes (c–e). In those three panels, the coloured surfaces represent areas of the trimer that are within 2 Å of α-1,2-mannosidase after docking the terminal mannoses on Man9GlcNAc2into the binding enzyme pocket, that is, clashes occur that impede enzyme access to its glycan substrates and are therefore predicted to prevent glycan processing. The variable loops V4 and V1 account for a large proportion of the clashes seen in panelsdande, respectively. The N262A mutation in particular showed a marked change in glycan processing, and this effect was replicated when the N262 site was deleted across a small cross-clade panel ( Supplementary Table 4 ). Reduced binding was also seen for the N262A and N386A mutants with a second conformation-dependent antibody, 17b, which also lost binding to the N130A mutant ( Fig. 3 ), presumably through alterations to the structure of the V1 loop [20] , [40] . These three mutants displayed greater levels of aggregation by western blotting ( Supplementary Fig. 4 ), supporting the hypothesis that they exhibit a degree of misfolding. Figure 3: Recognition of PNGS-deletion mutants by conformation-dependent antibodies. Binding of the conformation-dependent monoclonal antibodies b12 and 17b was tested against the panel of gp120 BaL PNGS-deletion mutants by capture ELISA. Error bars represent s.d. Each experiment was performed in duplicate and repeated three times. Full size image Misfolding of the N130A, N262A and N386A mutants could explain the disproportionately large changes observed in their glycan processing ( Fig. 1d ). In contrast, the significant changes observed for the N295, N339, N356, N392 and N448 mutants are likely to arise from disruption of glycan clusters leading to improved accessibility by ER and Golgi α-mannosidases. Effect of PNGS mutation of the N332 site of vulnerability A number of bnAbs have been isolated which incorporate the N332 glycan as part of their epitope. This so-called ‘supersite’ of immune vulnerability occupies a central location in the outer domain and lies within a high density of glycans ( Figs 4 and 5a ) [20] . Previous studies have indicated this site is occupied by oligomannose-type glycans [1] , [5] , [6] , suggesting that steric constraints restrict glycan processing at this site. To understand these steric constraints, we studied the location of the N332 glycan on the high-resolution BG505 SOSIP.664 trimer structure [21] and modelled how it would appear to α1,2-mannosidase, the enzyme that initiates glycan processing ( Fig. 4 ). The analysis was based on the glycan conformation of position N332 as revealed by the PGT128 co-crystal structure [17] . This revealed that the high density of glycans clustered around N332 provide significant steric constraints that impede access to the terminal mannose residues of N332 by α1,2-mannosidase. In addition to the constraints created by neighbouring glycans, the variable V1 and V4 loops, which project away from the trimer surface, may constitute additional obstacles ( Fig. 4c–e ). Figure 4: Steric barriers to the processing of Env glycans. The α-mannosidase enzyme has impeded access to the terminal sugars of the mannose patch due to steric constraints imposed by both protein and glycan moieties. ( a ) The high-resolution structure of α1,2-mannosidase (PDB accession code: 2RI9) bound to a disaccharide substrate shows how the substrate binds in a deep, concave pocket. ( b ) When the α-1,2-mannosidase structure is docked onto the surface of the HIV-1 Env trimer (hybrid model of EMD-5779 and PDB 3TYG) and aligned on the terminal D1, D2 or D3 arms of the Man 9 GlcNAc 2 moiety at position N332, there are significant clashes ( c – e ). In those three panels, the coloured surfaces represent areas of the trimer that are within 2 Å of α-1,2-mannosidase after docking the terminal mannoses on Man 9 GlcNAc 2 into the binding enzyme pocket, that is, clashes occur that impede enzyme access to its glycan substrates and are therefore predicted to prevent glycan processing. The variable loops V4 and V1 account for a large proportion of the clashes seen in panels d and e , respectively. 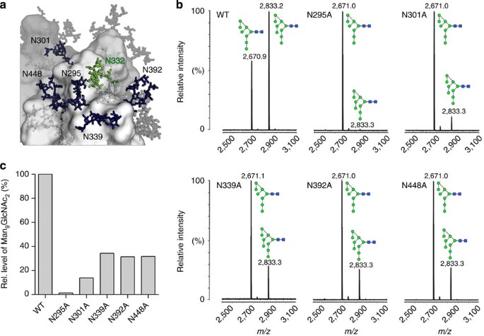Figure 5: The effect on processing at the N332 glycosylation site by the deletion of neighbouring glycans. (a) Model of the N332 glycan (green sticks) on the outer domain surrounded by neighbouring (dark blue sticks) and distant glycans (grey sticks). (b) Site-specific glycan analysis of the N332 site from a panel of mutants lacking the neighbouring glycans (Panela; dark blue glycans). A tryptic glycopeptide containing the N332 site (QAHCNLSR) was isolated and analysed by MALDI-MS to determine the glycoforms present. The same glycopeptide was analysed from gp120BaLmutants carrying PNGS-deletions proximal to N332. (c) Quantification of the abundance of Man9GlcNAc2on the wild-type and mutant glycopeptides as determined by MALDI-MS. Symbols as inFig. 2. Full size image Figure 5: The effect on processing at the N332 glycosylation site by the deletion of neighbouring glycans. ( a ) Model of the N332 glycan (green sticks) on the outer domain surrounded by neighbouring (dark blue sticks) and distant glycans (grey sticks). ( b ) Site-specific glycan analysis of the N332 site from a panel of mutants lacking the neighbouring glycans (Panel a ; dark blue glycans). A tryptic glycopeptide containing the N332 site (QAHCNLSR) was isolated and analysed by MALDI-MS to determine the glycoforms present. The same glycopeptide was analysed from gp120 BaL mutants carrying PNGS-deletions proximal to N332. ( c ) Quantification of the abundance of Man 9 GlcNAc 2 on the wild-type and mutant glycopeptides as determined by MALDI-MS. Symbols as in Fig. 2 . Full size image The high density of glycans in this region raises the question of what effect loss of nearby glycans could have on the processing of the N332 glycan and, importantly, how this may affect recognition by bnAbs. To address this, a tryptic glycopeptide containing the N332 site (QAHCNLSR) was isolated by reverse-phase high-performance liquid chromatography (RP-HPLC) fractionation and analysed by matrix-assisted laser desorption/ionization-mass spectrometry (MALDI-MS) to determine the glycoforms present. The MALDI-MS/MS spectrum of the glycopeptide is shown in Supplementary Fig. 5a . Consistent with its structurally constrained location and previous studies, the glycan structures identified at this site were found to be exclusively Man 8 GlcNAc 2 and Man 9 GlcNAc 2 , with 35 and 65% abundances, respectively ( Fig. 5b,c ). No smaller oligomannose structures or complex-type glycans were detected. The reproducibility of this method is demonstrated in Supplementary Fig. 5b . To determine whether nearby sites played a role in determining the glycan structures present at N332, the same tryptic glycopeptide was purified and analysed from the N301A, N295A, N339A, N392A and N448A mutants. The MALDI mass spectra of these profiles demonstrated an altered distribution of glycoforms, with Man 9 GlcNAc 2 being lost in favour of Man 8 GlcNAc 2 ( Fig. 5b,c ). In line with its close proximity to N332, loss of the N295 glycan was found to have the largest impact on processing at the N332 site, resulting in an almost complete conversion of Man 9 GlcNAc 2 to Man 8 GlcNAc 2 . Loss of the N301 glycan, which reaches over the gp120 surface towards N332, also caused a distinct loss of Man 9 GlcNAc 2 at the N332 site, and smaller changes were also observed for the N339A and N392A mutants. It is likely that the influence of the N448 glycan is mediated through the N295 glycan with which it is clustered. These observations demonstrate that the environment of a glycan is important in modulating its level of processing. However, at least for the N332 site, the density of surrounding glycans is sufficiently high to act as a buffer for single PNGS-deletions, limiting the effect on processing to minor re-distributions in oligomannose-type structures. To determine whether changes to the glycan shield observed upon glycosylation site deletion could affect antibody recognition, the panel of gp120 BaL PNGS-mutants was screened for binding to the N332-dependent bnAbs: 2G12, PGT121, PGT128 and PGT135 ( Fig. 6 ; Supplementary Table 3 gives the IC 50 values). Consistent with previous reports [13] , [15] , [41] , [42] , 2G12 binding was reduced in the N332A, N295A, N386A and N392A mutants. The loss of N295 and N392 were found to be most detrimental to binding, and these glycans have been shown in a 2G12 Fab 2 complex with HIV Env to bind within the conventional V H /V L binding site [42] . Interestingly, the effect of the N332-knockout was very modest, and this glycan was shown to bind within the novel secondary V H /V H ′ interface formed by domain exchange in the complex. The loss of N332 was tolerated less well by the PGT antibodies with deletion of known secondary sites also causing reduced binding. Binding by PGT121, which recognizes both oligomannose- and complex- type glycans [19] , [26] , was robust across the remaining panel of mutants with the exception of N262A and N130A which, as discussed above, is a likely consequence of altered protein conformation. Interestingly, the observation that N386A mutation retained binding to PGT121 indicates that perturbations in folding may be localized. In contrast, PGT128 binding appeared to be modestly reduced upon loss of the N295, N386 and N392 sites, which were not contacted by PGT128 in the crystal structure of the antibody–eODmV3 complex [17] . Glycan array data, and the extensive contacts made by PGT128 with the terminal mannose residues of the D1 and D3 arms, support a preferred specificity for Man 8 GlcNAc 2 and Man 9 GlcNAc 2 glycans. The decrease in PGT128 binding upon mutation of the N295, N386 and N392 sites may be due to changes in glycan processing or flexibility at the N332/N301 epitope. The observation that N295A retains Man 8 GlcNAc 2 glycans at N332 ( Fig. 5 ) suggests a role for changes in glycan flexibility for this mutant or altered processing at N301. 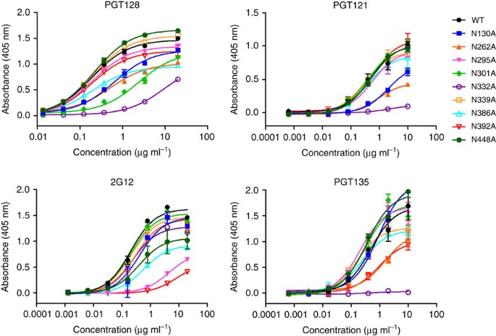Figure 6: Recognition of glycan site deletion mutants by N332-specific bnAbs. Binding of a panel of N332-specific bnAbs, including 2G12, PGT128, PGT135 and PGT121, was tested against the panel of gp120BaLglycan site deletion mutants by capture ELISA. Error bars represent s.d. Each experiment was performed in duplicate and repeated three times. Figure 6: Recognition of glycan site deletion mutants by N332-specific bnAbs. Binding of a panel of N332-specific bnAbs, including 2G12, PGT128, PGT135 and PGT121, was tested against the panel of gp120 BaL glycan site deletion mutants by capture ELISA. Error bars represent s.d. Each experiment was performed in duplicate and repeated three times. Full size image Binding of PGT135 was significantly reduced in the N332A and N392A mutants, consistent with their observed roles in antibody binding [20] . Loss of the N295 site, which has been found to be important in a strain-dependent manner, was tolerated in gp120 BaL , although loss of N386 slightly decreased binding. In addition, the N339 glycan was also implicated in formation of the PGT135 epitope, either directly or indirectly ( Fig. 6 ). Glycan array data for PGT135, and neutralization of pseudovirus with altered glycosylation profiles, suggest that there is a preference for Man 7 GlcNAc 2 and Man 8 GlcNAc 2 glycans at certain sites. Therefore, removal of bystander glycan sites that impact the oligomannose structures within the PGT135 epitope could impact binding [20] . Overall, these results show that processing of gp120 glycans are influenced by their environment, with removal of neighbouring sites influencing the abundance of different glycan structures present. Such bystander effects were observed at the N332 site, which could explain the dependence of some bnAbs on additional glycan sites not thought to be directly contacted by bnAbs. Effect of PNGS deletion on virus neutralization To test the impact of glycan site removal on glycan processing in the context of the HIV-1 envelope trimer, we made several BaL pseudoviruses, each with a single PNGS removed (N130, N262, N295, N301, N332, N386 and N392). The impact of these glycan deletions on neutralization by our panel of N332-dependent bnAbs and b12 was then analysed ( Fig. 7 ). Neutralization by b12 was unaffected for the N130A, N295A, N332A and N392A mutants. However, the N301A and N386A mutants displayed increased sensitivity, consistent with previous observations that removal of these glycans exposes the CD4bs [3] . An increased sensitivity was also observed for the N262A mutant, which could similarly arise from local changes in protein conformation increasing accessibility to the CD4bs. The N262A mutant was also more sensitive to several of the N332-dependent bnAbs, indicating increased accessibility of these epitopes. The effects of the N130A mutation on neutralization were subtler than observed for the gp120 monomer binding, possibly reflecting differences in the assays or, conceivably, the differences in the presentation of that site between monomeric gp120 and virion-associated gp120. However, reduced plateaus were observed for PGT128 and PGT130, which could be a consequence of either altered epitope conformation or glycosylation composition. 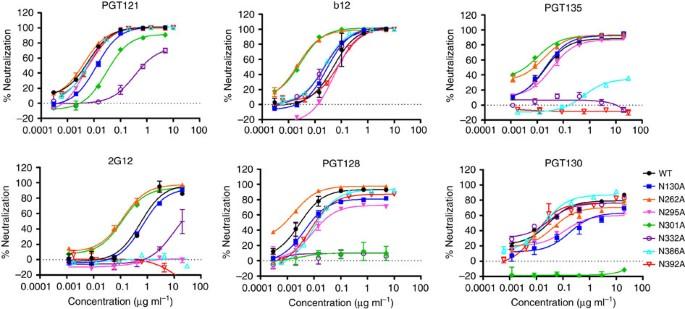Figure 7: The effect of glycan site deletion on neutralization by N332-specific bnAbs. Neutralization of the BaL wild-type virus and mutant viruses by b12 and N332-specific bnAbs, including PGT121, PGT135, 2G12, PGT128 and PGT130. Error bars represent s.d. Each experiment was performed in duplicate and repeated three times. Figure 7: The effect of glycan site deletion on neutralization by N332-specific bnAbs. Neutralization of the BaL wild-type virus and mutant viruses by b12 and N332-specific bnAbs, including PGT121, PGT135, 2G12, PGT128 and PGT130. Error bars represent s.d. Each experiment was performed in duplicate and repeated three times. Full size image Loss of glycan sites known to form bnAb epitopes resulted in reduced neutralization (for example, N332A for PGT128 and 2G12, N301A for PGT128 and PGT130, N295A for 2G12, N386A for 2G12 and PGT135, and N392A for 2G12 and PGT135). The N332A mutation had a more limited impact on neutralization by PGT130 and PGT121, arising from the ability of these bnAbs to bind adaptably to the mannose patch and utilize alternative glycans in the absence of the N332 glycan [27] . Interestingly bnAbs PGT128, PGT130 and PGT135 were unable to neutralize the wild-type virus to 100%, which could indicate the presence of glycoforms that they are unable to bind. In contrast, PGT121, which has been shown to recognize both complex- and oligomannose-type glycans [19] , [26] , was able to neutralize 100% of the wild-type virus. The N295A mutation was tolerated to varying degrees by the bnAbs, and broadly correlated with the results of the gp120 monomer; neutralization by PGT121 and PGT135 was maintained, while reduced plateaus were observed for PGT128 and PGT130. With the emergence of a large number of glycan-reactive bnAbs, it has become apparent that the ‘non-self’ oligomannose patch within gp120 represents an immunogenic region that could be exploited for vaccine design [32] . This study has demonstrated the persistence of the oligomannose population in the face of glycan-site deletion, which, given the shifting nature of the HIV-1 glycan shield [33] , [34] , is an important requirement for ensuring the breadth and potency of a bnAb response. The minimal disruption to processing observed upon deletion of PNGSs suggests that the density of glycans on gp120, is sufficiently high to tolerate individual losses. However, it remains to be determined whether there is a critical number of deletions that would reduce the density sufficiently to trigger a larger-scale conversion of oligomannose-type glycans to complex-type glycans, and whether or not this is a realistic prospect in native virus given that many sites bearing oligomannose glycans are highly conserved ( Fig. 1b,c ). It is possible that this answer may vary between different isolates, depending on their base level of glycan density. It is also important to note that additional glycan–glycan and glycan–protein interactions exist within the context of the trimer. By using monomeric gp120, we have focused our study on the integrity of the intrinsic mannose patch of the outer domain. Given the structural similarity of the outer domain in the context of monomer and trimer, and the conservation of the epitopes of many glycan-dependent antibodies, we suggest that there are also shared rules governing the formation of the intrinsic-mannose patch in monomers and trimers. Although the precise structural factors shaping the formation and stability of trimer glycosylation requires investigation [7] , [8] , we predict that trimerization will only serve to further stabilize glycan processing. A number of the best characterized glycan-binding bnAbs to date have been found to specifically target the N332 glycan [9] , [17] , [19] , [20] , [21] , although it is now believed that the area of vulnerability extends across Env [11] , [12] , [16] , [24] , [25] , [43] . However, N332 is central to the intrinsic mannose patch and we therefore focused our analysis of PNGS-deletions on the processing of glycoforms at the N332 site, and the consequences for bnAb binding and neutralization. The removal of a single glycan site was found to have a very modest effect on the glycan structures at the N332 site, and this was reflected in the apparent tolerance of a panel of N332-dependent bnAbs to these mutations. The glycan at the N295 site, which, when deleted, had the biggest impact on N332 glycan-processing, was an exception. The reduced neutralization displayed by PGT128 and PGT130, which do not directly recognize the N295 glycan, most likely reflects a more widespread perturbation in glycan processing to structures exhibiting reduced antibody binding. These results provide several important considerations for vaccine design. First, a question that remains to be answered relates to whether a successful immunogen should contain epitopes bearing a more restricted population of glycan structures, to generate the most potent response possible, or whether the presence of a more diverse selection of glycoforms would promote a polyclonal response that offers increased breadth. A better understanding of the glycan specificity of bnAbs would help to address this question, as well as site-specific glycan analysis of the functional envelope spike. Secondary to this, it is important to consider how to generate the desired glycoforms on a site-specific basis. Data presented here suggest that to reproduce the target epitopes in an immunogen context, it will be necessary to consider the wider environment of the key glycan sites, particularly for oligomannose sites that depend on a high density of glycans to restrict glycan processing. This study has highlighted important regions of glycan–glycan packing that contribute to maintenance of the oligomannose population, and it is likely that their presence will be necessary to reproduce it in an immunogen context. Our results demonstrate that the presence or absence of individual sites can regulate the precise type of oligomannose structures produced. For example, the levels of the Man 9 GlcNAc 2 were found to be particularly sensitive to PNGS-deletion, and thus with careful immunogen design it may be possible to precisely fine-tune the degree of glycoform heterogeneity at relevant sites. One site of note that could emerge as a site of vulnerability is N262 as it is almost 100% conserved ( Fig. 1c ) and has been shown to be occupied by oligomannose-type glycans [1] , [37] . Previous studies involving knockout of this glycan have shown it has an important role for infectivity [10] , [44] , [45] , [46] . While our BaL N262A pseudovirus was still infectious, increased sensitivity to b12 neutralization was indicative of an altered protein conformation, which was supported by observations of the recombinant N262A gp120 BaL . In the crystal structure of the BG505 SOSIP.664 trimer [21] , the N262 glycan makes extensive contacts with the protein backbone, rationalizing both its protection from endoglycosidase cleavage and its occupation by oligomannose-type glycans. Such a stabilizing role was also observed in a more recent structure of fully glycosylated gp120 monomer [47] . Oligomannose-type glycans have previously been reported in sites that are inaccessible to glycosidases [48] , [49] , and under-processed glycans often contribute to protein fold stability [50] . The requirement of this glycan is also highlighted by studies with antiviral carbohydrate-binding agents such as cyanovirin-N and Griffithsin, which target oligomannose-type glycans. Resistance profiling with these agents consistently selects for PNGS-deletion mutants, which mostly map to sites known to contain oligomannose glycans including N332, N295, N339, N386, N392 and N448; however, deletion of N262 is rarely observed [51] , [52] , [53] , [54] , [55] . The presence of oligomannose-type glycans on Env has consequences beyond antibody recognition, for example through their interactions with cellular receptors of the immune system. One of the best characterized interactions occurs with the dendritic cell-specific intercellular adhesion molecule-3 (ICAM)- grabbing non-integrin (DC-SIGN) receptor on DCs in the mucosal tissues, which facilitates the trans-infection of CD4 + CCR5 + T cells in secondary lymphoid tissues [56] , [57] , [58] . However, more relevant, perhaps, from a vaccine design perspective are observations that oligomannose-type glycans can induce secretion of the immunosuppressive cytokine, IL-10, through interaction with receptors on monocyte-derived DCs [59] . Such an interaction may contribute to the poor immunogenicity of HIV-1 Env as a vaccine candidate, and indeed it has been shown that enzymatic removal of gp120 mannose residues, or occlusion using Griffithsin, improves the immunogenicity of recombinant gp120 (refs 60 , 61 ). Thus, an effective vaccine strategy may have to balance the requirement for faithful replication of bnAb epitopes with the immunogenic properties of vaccine candidates. In summary, we have shown that the conservation of the oligomannose patch, and its resilience in the face of glycan-site deletion, makes it a robust target for vaccine design. Multiple bnAbs have been isolated that display subtly different, yet overlapping, epitopes within this region, suggesting that the induction of a polyclonal response against it would protect against a diverse viral swarm. Furthermore, data presented here on the persistence of the mannose patch provide important insights for the design of future candidate immunogens. Site-directed mutagenesis The cloning of gp120 BaL into the pHLsec expression vector has previously been described [62] . Individual knockout of all 23 PNGSs of BaL gp120 was performed by mutating asparagines (within the sequence Asn-X-Ser/Thr, where X is any amino acid except proline) to alanine. Mutagenesis was performed by the overlap extension PCR method [63] , using ∼ 1 ng of WT pHLsec.BaL as the template DNA. A list of primers used is given in Supplementary Table 5 . The full Env sequence for each construct was verified by DNA sequencing. Mutations in the full-length envelope were made using site-directed mutagenesis and the sequences were verified by DNA sequencing. A list of primers used is given in Supplementary Table 6 . Protein expression and purification Human embryonic kidney (HEK) 293T cells were purchased from the American Type Culture Collection and maintained in Dulbecco’s Modified Eagle’s Medium containing 10% fetal bovine serum, 50 U ml −1 penicillin, and 50 μg ml −1 streptomycin. Recombinant gp120s were expressed under serum-free conditions, by transient transfection of expression plasmids using polyethylenimine (PEI) in a PEI:DNA ratio of 3.5:1 (w/w). Comparable mutants were expressed in parallel to avoid variation arising from fluctuating cell culture conditions. Transfected cultures were incubated for 3 days before supernatants were harvested and filtered through a 0.22-μM membrane (Millipore). Gp120 was purified by immobilized metal affinity chromatography using a HisTrap HP column (GE Healthcare) according to the manufacturer’s instructions. Eluted fractions were concentrated using 50 kDa cutoff centrifugal spin filters (Vivaspin). Enzymatic release of N-linked glycans N-linked glycans were released from gp120 in-gel using PNGase F (New England Biolabs). His-purified gp120 was resolved by SDS–PAGE and stained with Coomassie Blue. Following destaining, the band corresponding to monomeric gp120 was excised and washed extensively with acetonitrile and water. Gel bands were then incubated with PNGase F for 16 h at 37 °C, following manufacturer’s instructions. Released glycans were eluted from the gel with water and dried in a SpeedVac concentrator. Fluorescent labelling of N-linked glycans Released glycans were subsequently fluorescently labelled and purified as previously described [64] . In brief, dried glycans were resuspended in 30 μl water before addition of 80 μl labelling mixture (comprising 30 mg ml −1 2-aminobenzoic acid [2-AA] and 45 mg ml −1 sodium cyanoborohydride in a solution of sodium acetate trihydrate [4% w/v] and boric acid [2% w/v] in methanol). Samples were incubated at 80 °C for 1 h then allowed to cool. Excess label was removed using Spe-ed Amide-2 cartridges. HILIC-UPLC analysis of N-linked glycans Fluorescently labelled glycans were separated by HILIC-UPLC using a 2.1 mm × 10 mm Acquity BEH Amide Column (1.7 μm particle size; Waters, Elstree, UK). The following gradient was run: time=0 min ( t =0): 22% A, 78% B (flow rate of 0.5 ml min −1 ); t =38.5: 44.1% A, 55.9% B (0.5 ml min −1 ); t =39.5: 100% A, 0% B (0.25 ml min −1 ); t =44.5: 100% A, 0% B; t =46.5: 22% A, 78% B (0.5 ml min −1 ), where solvent A was 50 mM ammonium formate, pH 4.4, and solvent B was acetonitrile. Fluorescence was measured using an excitation wavelength of 330 nm and a detection wavelength of 420 nm. Difference plots were generated in MATLAB (The MathWorks). Enzymatic digestion of released glycans The abundance of oligomannose glycans was measured by digestion with Endoglycosidase H, which cleaves oligomannose-type glycans but not complex-type glycans (Endo H; New England Biolabs). 2-AA labelled glycans were resuspended in water and digested with Endo H for 16 h at 37 °C, according to the manufacturer’s instructions. Digested glycans were cleaned using a PVDF protein-binding membrane plate before HILIC-UPLC analysis. The abundance of oligomannose-type glycans was calculated, as a relative percentage, by integration of the HILIC-UPLC chromatograms before and after Endo H digestion, following normalization. The magnitude of change was calculated as a % change in abundance, relative to wild-type. Structural modelling of glycosylated Env A model of the BaL gp120 trimer was constructed using the recently solved atomic-level resolution structure of a BG505 SOSIP.664 gp140 trimer (PDB accession code: 4NCO) [21] . First, atomic clashes present in the 4NCO crystal structure were relieved and missing side-chains rebuilt, by executing 1,000 symmetric ROSETTA-fixbb simulations, selecting the lowest scoring model, and then running a constrained ROSETTA-relax simulation. Next, the BaL sequence was modelled onto the gp120 trimer structure, by running 1,000 ROSETTA-remodel trajectories [65] , which included building new conformations for the variable loops, and then filtering the models by structural metrics. The best 15 models were considered as an ensemble of possible BaL gp120 trimer structures, as each model was in the top 33% of the three structural metrics Ramachandran (rama), attractive portion of the Lennard-Jones potential (fa_atr) and the total ROSETTA score. Each N-linked glycosylation motif for each of the 15 models was decorated with Man 8 GlcNAc 2 glycans at sites of predicted oligomannose-type glycans and with Man 5 GlcNAc 2 glycans at remaining sites. GlycanRelax [66] was used to approximate the conformational behaviour of glycans in a glycoprotein context. For each model, 10 separate GlycanRelax trajectories of 10,000 cycles of MonteCarlo trials were carried out. Each glycan on the gp120 was allowed to move independently throughout the GlycanRelax minimization. A single low energy model was chosen for the figures. Purification of an N332 glycopeptide Gp120 was resolved by SDS–PAGE, and the monomer excised and washed as described above. Reduction was carried out by addition of 10 mM Dithiothreitol in 100 mM ammonium bicarbonate and incubation at 65 °C for 30 min. Alkylation was subsequently performed by addition of 50 mM Iodoacetamide in 100 mM ammonium bicarbonate, with incubation at room temperature for 50 min. Trypsin (Promega) was then added at a concentration of 12.5 μg ml −1 and incubated at 37 °C for 16 h. Glycopeptides were eluted from the gel with alternate washes of water and acetonitrile, filtered through a 0.45 μM membrane (Whatman), and dried in a SpeedVac concentrator. After resuspension in 0.1% TFA, the glycopeptide pool was fractionated by reverse phase-HPLC using a Jupiter C18 5 μm 250 × 4.5 mm column (300 Å pore size) (Phenomenex) and a Dionex U3000 LC system. The following gradient was run at a flow rate of 1 ml min −1 , with fractions being collected every minute for 90 min: time=0 min ( t =0): 95% A, 5% B; t =5: 95% A, 5% B; t =90: 10% A, 90% B; t =95: 10% A, 90% B; t =97: 95% A, 5% B; t =120: 95% A, 5% B, where solvent A was 50 mM ammonium formate, pH 4.4, and solvent B was acetonitrile. UV absorbance was detected at 214 and 280 nm. Mass spectrometric analysis of glycopeptides Glycopeptide fractions were desalted using C18 ZipTip pipette tips, according to the manufacturer’s instructions, before spotting onto a ground steel target plate in a solution of 10 mg ml −1 2,5-Dihydrozybenzoic acid in 50% acetonitrile. MALDI-MS was performed using an Autoflex Speed MALDI-TOF/TOF instrument (Bruker), operated in positive ion mode. MS/MS was performed to confirm the peptide identity. ELISA Antibodies b12, 17b, 2G12, PGT121, PGT128 and PGT135 were obtained from the International AIDS Vaccine Initiative (IAVI, New York, NY). Microtitre ELISA plates (Corning) were coated with mouse anti-HIS capture antibody (2 μg ml −1 in PBS; Life Technologies) overnight at 4 °C. Plates were washed five times with a solution of PBS containing 0.05% Tween 20 (v/v) and then blocked for 1 h at room temperature with 5% non-fat milk in PBS+0.05% Tween (blocking buffer). Gp120 was then added at a concentration of 2 μg ml −1 in blocking buffer, followed by incubation for 1 h at room temperature. Plates were washed ( × 5) before addition of primary antibodies (b12, 17b, 2G12, PGT121, PGT128 & PGT135). A 1:5 dilution series was used starting at 20 or 40 μg ml −1 in blocking buffer. Incubation was carried out at room temperature for 2 h. Plates were then washed ( × 5) and alkaline phosphatase-conjugated goat anti-human Fab secondary antibody (Thermo Scientific Pierce) was added as a 1:1,000 dilution in blocking buffer. Plates were washed ( × 5) and then AP substrate (50 μl per well) was added. The OD at 405 nm was measured after 20 min. Virus neutralization assay To produce pseudoviruses, plasmids encoding Env were co-transfected with an Env-deficient genomic backbone plasmid (pSG3ΔEnv) in a 1:2 ratio with the transfection reagent PEI (1 mg ml −1 , 1:3 PEI:total DNA, Polysciences) into HEK 293T cells. Pseudoviruses were harvested 72 h post transfection for use in neutralization assays [67] . Neutralizing activity was assessed using a single round replication pseudovirus assay with TZM-bl target cells, as described previously [68] . In brief, TZM-bl cells were seeded in a 96-well flat bottom plate at a concentration of 20,000 cells per well. The serially diluted antibody/virus mixture, which was pre-incubated for 1 h, was then added to the cells and luminescence was quantified 72 h following infection via lysis and addition of Bright-Glo Luciferase substrate (Promega). To determine IC 50 values, serial dilutions of mAbs were incubated with wild-type virus or mutant virus and the dose–response curves were fitted using nonlinear regression. How to cite this article: Pritchard, L. K. et al. Glycan clustering stabilizes the mannose patch of HIV-1 and preserves vulnerability to broadly neutralizing antibodies. Nat. Commun. 6:7479 doi: 10.1038/ncomms8479 (2015).